Prevailing oxic environments in the Pacific Ocean during the mid-Cretaceous Oceanic Anoxic Event 2 The occurrence of Oceanic Anoxic Event 2 (OAE2) 94 million years ago is considered to be one of the largest carbon cycle perturbations in the Earth's history. The marked increase in the spatial extent of the anoxic conditions in the world's oceans associated with OAE2 resulted in the mass accumulation of organic-rich sediments. Although extensive oceanographic studies of OAE2 have been undertaken in the Atlantic Ocean, the Tethys Sea, and the epicontinental seas of Europe and America, little is known about OAE2 in the Pacific Ocean. Here, we present high-resolution carbon-isotope and degree of pyritization (DOP) data from marine sequences that formed along the continental margins of North America and Asia below the northeastern and northwestern Pacific Ocean. The predominance of low DOP values in these areas revealed that the continental margins of the Pacific Ocean were oxic for most of the OAE2 interval. The mid-Cretaceous Oceanic Anoxic Event 2 (OAE2), which occurred near the Cenomanian/Turonian boundary, is one of the most prominent perturbations in the carbon and sulphur cycles in the Earth's history. The expansion of the anoxic environment in the oceans due to the increase in primary production is considered to have resulted in the widespread deposition of organic-rich sediments (so-called 'black shales') and the mass extinction of marine fauna [1] , [2] . Numerous studies have clarified the detailed palaeoceanographic and faunal changes across OAE2 in parts of the Atlantic Ocean, Tethys Sea and the epicontinental seas of Europe and America. Several of these studies have demonstrated that anoxic environments expanded from the photic zone to depths of ∼ 3,500 m (refs 3 , 4 ), and that significant faunal and environmental turnover occurred across OAE2 (ref. 2 ). Recent hypotheses support the view that the ultimate trigger for OAE2 was large scale volcanic activity, which stimulated primary production by enhancing nutrient flux and recycling [5] , [6] , [7] . A likely area for this volcanic activity is the Caribbean Plateau [7] , [8] , but other episodes of contemporaneous volcanism, such as that associated with the Kerguelen Plateau, the Ontong Java Plateau and the Madagascar flood basalt, are also possible candidates [9] , [10] ( Fig. 1 ). 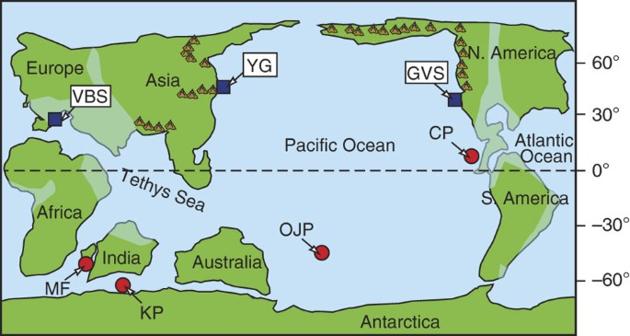Figure 1: Palaeogeography and study areas 90 Myr ago. Blue squares show study areas and the reference section of the OAE2 in France. Red circles represent the location of the large igneous provinces that erupted during OAE2. GVS, Great Valley Sequence; CP, Caribbean Plateau; KP, Kerguelen Plateau; MF, Madagascar Flood Basalt; OJP, Ontong Java Plateau; VBS, Vocontian Basin Sequence; YG, Yezo Group. Figure 1: Palaeogeography and study areas 90 Myr ago. Blue squares show study areas and the reference section of the OAE2 in France. Red circles represent the location of the large igneous provinces that erupted during OAE2. GVS, Great Valley Sequence; CP, Caribbean Plateau; KP, Kerguelen Plateau; MF, Madagascar Flood Basalt; OJP, Ontong Java Plateau; VBS, Vocontian Basin Sequence; YG, Yezo Group. Full size image The Pacific Ocean constituted more than 60% of the world's ocean during the mid-Cretaceous and was characterized by extensive volcanism in the Caribbean and Ontong Java plateaus during OAE2 ( Fig. 1 ). Nonetheless, despite the importance of the Earth's ocean–climate system, few attempts have been made to accurately characterize the palaeoceanographic changes and the distributions of black shales across OAE2 in the Pacific Ocean except for a few pioneer works [11] , [12] . The relative lack of research in this area is primarily because most of the Cretaceous oceanic crust in the Pacific Ocean has been subducted under continents. This subduction has resulted in poor recoveries of Cretaceous sediments from the Ocean Drilling Program and Deep Sea Drilling Program cores obtained at these sites and has complicated the identification the OAE2 horizon. In this study, to accurately clarify the detailed palaeoceanographic changes across OAE2 in the Pacific Ocean, assessments of the micropalaeontology, degree of pyritization (DOP) and carbon-isotope analyses of wood fragments were performed on OAE2-interval sediments from the Budden Canyon Formation comprising the Great Valley Sequence (GVS) that crops out in northern California as well as the Saku Formation of the Yezo Group (YG), which crops out in central Hokkaido, Japan. Our results indicate that the continental margins of the Pacific Ocean were oxic for most of the OAE2 interval because of the predominance of low DOP values in these study areas. Geological settings and lithofacies The GVS accumulated at ∼ 30–40° N along the North American active continental margin in the northeastern Pacific Ocean [13] , and the YG at ∼ 45° N along the Asian active continental margin in the northwestern Pacific Ocean ( Fig. 1 ) [14] , [15] . Previous studies on benthic foraminifera reported that both strata were formed at upper bathyal depths [16] , [17] , which are usually characterized by the development of oxygen minimum zones (OMZs) [18] . The upper Cenomanian–lower Turonian strata of the GVS and YG consist primarily of mudstone and muddy sandstone with intercalations of thin- to very thick-bedded turbidite sandstone and felsic tuff ( Fig. 2 ). Marine macro- and microfossils have been found in all of the strata in these sequences, which also contain small gastropod and radiolarian fossils derived from flood events in the upper OAE2 intervals in the GVS and YG, respectively ( Fig. 2a,b ). Whereas neither of the strata were intercalated with the so-called 'black shales' and organic carbon-rich sediments, both exhibit varying degrees of bioturbation throughout the OAE2 interval. Although the total organic carbon (TOC) content of both strata ranged from 0.5 to 1.5%, most of the organic matter is derived from terrestrial plants [11] , [17] . Mean sedimentation rates across the OAE2 intervals were estimated to be 30.5–31.9 cm ky −1 in the GVS and 14.8–15.5 cm ky −1 in the YG, which is several tens to hundreds of times greater than the hemipelagic and pelagic sediments that accumulated along the passive continental margin of the Atlantic Ocean and the Tethyan Sea [19] , [20] . 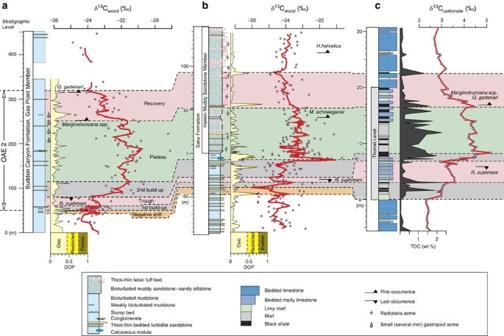Figure 2: Stratigraphic columns and geochemical and biostratigraphic results for the two studied sites and one reference site. (a) Great Valley Sequence (GVS) at California, USA, (b) the Yezo Group (YG) in Hokkaido, Japan and (c) Vocontian Basin Sequence (VBS) in Provence, France. Closed pink circles represent the carbon-isotope values of wood and carbonate. (a) and (b) Five-point moving average for the carbon isotopes of wood (red lines). (c) Carbon-isotope curve for carbonate rocks (red line). Degree of pyritization (DOP) and total organic carbon (TOC) content are represented by the yellow and black area graphs, respectively. Lithology, carbon isotope and TOC data of the section graph (c) are from ref.20. Parts of bio-events are from ref.24. Figure 2: Stratigraphic columns and geochemical and biostratigraphic results for the two studied sites and one reference site. ( a ) Great Valley Sequence (GVS) at California, USA, ( b ) the Yezo Group (YG) in Hokkaido, Japan and ( c ) Vocontian Basin Sequence (VBS) in Provence, France. Closed pink circles represent the carbon-isotope values of wood and carbonate. ( a ) and ( b ) Five-point moving average for the carbon isotopes of wood (red lines). ( c ) Carbon-isotope curve for carbonate rocks (red line). Degree of pyritization (DOP) and total organic carbon (TOC) content are represented by the yellow and black area graphs, respectively. Lithology, carbon isotope and TOC data of the section graph ( c ) are from ref. 20 . Parts of bio-events are from ref. 24 . Full size image Biostratigraphy A detailed bio- and carbon isotope-stratigraphic framework across the OAE2 interval has been determined for Pueblo (USA), Eastbourne (England), Tarfaya (Morocco), Wadi Bahloul (Tunisia), Provence (France) and Gubbio (Italy) [19] , [20] , [21] , [22] , [23] . These studies have revealed a detailed stratigraphic range of age-diagnostic marker species in macro- and microfossils across OAE2. Although we were unable to obtain age-diagnostic macrofossils, several planktic foraminiferal and calcareous nannofossil marker species were obtained from the GVS and YG. Rotalipora cushmani (Morrow), which is a commonly used Upper Cenomanian planktic foraminiferal marker species, occurs intermittently up to the 80 m level in the GVS ( Fig. 2a ) and the −30 m level in the YG ( Fig. 2b ). The last occurrence of R. cushmani is correlated with the uppermost Cenomanian, which is equivalent to the basal horizon of the OAE2 interval ( Fig. 2c ) [19] , [20] , [21] , [22] , [23] . The first occurrence of the calcareous nannofossil marker species Quadrum gartneri Prins and Perch-Nielsen, which occurs at the base of the Turonian and the upper part or just above the OAE2 interval ( Fig. 2c ) [19] , [20] , [21] , was at the 315 m level in the GVS ( Fig. 2a ). However, we were unable to identify this species in the YG because calcareous nannofossils were both poorly represented and preserved in the Hakkin Muddy Sandstone Member. Although we were unable to obtain Turonian planktic foraminiferal marker species from the studied interval in the YG, previous studies have reported the first occurrence of Marginotruncana schneegansi (Sigal) and Helvetoglobotruncana helvetica (Trujillo) to be 42 and 116 m levels in this section, respectively [11] , [24] ( Fig. 2b ). The first occurrence of M. schneegansi is thus placed at the uppermost horizon of the OAE2 interval [22] , [23] and that of H. helvetica at the uppermost part, or just above the OAE2 interval [19] , [20] , [21] , [22] , [23] in the Tethyan realms. Consequently, both bio-events are correlated with the lower Turonian. Carbon-isotope stratigraphy As organic carbon preferentially sequesters isotopically light carbon, episodes of increased organic carbon burial are recorded as positive excursions in the stable carbon isotope ratios (δ 13 C) of both carbonates and organic carbon in the geological record. Conversely, a negative δ 13 C shift is generally associated with an increase in emissions of volcanic CO 2 , methane hydrate decomposing, weathering of organic matter and carbonate burial [25] . The levels of δ 13 C during OAE2 are characterized by two positive peaks punctuated by a small trough, which is a smaller peak followed by a second, broad trapezoidal peak. Such δ 13 C patterns, which have been reported at several disparate sites [21] , can be divided into five phases in the following ascending order: the first build-up, a trough, the second build-up, a plateau and a recovery [26] . The δ 13 C values and five-point moving averages obtained for bulk wood fragments from the GVS and YG across OAE2 are shown in Figure 2a,b . The results of the δ 13 C wood values are stratigraphically very scattered, which may have arisen because of vital or diagenetic effects, changes in the climate or the hydrological cycle on land. However, the five-point moving average curves of δ 13 C wood and the biostratigraphic data from the GVS and YG are correlated well with the δ 13 C carbonate curve and the biostratigraphy of the Vocontian Basin Sequence (VBS) ( Fig. 2 ). In addition, the δ 13 C wood curves could be divided into five phases, from the first build-up to recovery phases. Although the boundaries of each δ 13 C phase could not be defined clearly because of marked fluctuations in the δ 13 C wood values throughout the sequences, the overall similarity in δ 13 C curves of wood fragments between the Pacific sections (GVS and YG) and marine carbonates from the VBS demonstrates that global terrestrial and marine carbon cycles were closely coupled during OAE2. Conversely, no such coupling was observed for the δ 13 C curve of carbonate and wood for which a prominent negative δ 13 C excursion was observed at the base of the first build-up phase in the GVS (43–50 m level in Fig. 2a ) and YG (−47 to −39 m level in Fig. 2b ), but not in the VBS ( Fig. 2c ). This negative shift is referred to here as the negative excursion phase. Degree of pyritization The DOP, which is the ratio of the iron in pyrite to the total amount of iron in the sediments, is considered to be a reliable indicator of the redox condition (or dissolved oxygen levels) of bottom water because much of the pyrite in sedimentary environments arises from the microbial reduction of sulphates [27] . The following guidelines were developed to characterize the DOP in sediments: DOP<0.45 indicates oxic bottom-water conditions, 0.45<DOP<0.75 indicates 'restricted' bottom-water conditions and DOP>0.75 indicates 'inhospitable' (euxinic) bottom-water conditions [27] . However, to obtain accurate results, the sediments used for DOP measurements must contain sufficient iron-containing clastic materials, because sediments consisting primarily of biogenic materials (for example, limestone and chert) are unsuitable for DOP analysis [27] . Although the sedimentary rocks of the VBS are mainly composed of calcareous fossils that are not suitable for DOP analysis, the sediments of the GVS and YG consist mainly of terrigenous detritus, which is well suited to the measurement of DOP. Our DOP analysis revealed that most of the OAE2 intervals in the GVS and YG strata had oxic bottom-water conditions with DOP values <0.45 ( Fig. 2a,b ). These findings support the observation that bioturbations and benthic foraminifera occur throughout the OAE2 interval in both strata ( Fig. 2 ). However, higher DOP values (>0.45) briefly occur at five horizons in the GVS (45, 50, 55, 110 and 265 m levels, Fig. 2a ), and at four horizons in the YG (−46 m, −16 to −15 m, −5 to −2 m and 57 m levels, Fig. 2b ). It is noteworthy that the DOP peaks in the negative shift and basal recovery phases appear to be synchronous between the GVS and YG. These high DOP horizons are characterized by decreased bioturbation intensity, an increase of 0.2–0.5% in TOC values, and a predominance of dysoxic benthic foraminiferal taxa [17] . The presence or absence of negative δ 13 C excursions at the base of the OAE2 boundary have been examined extensively [8] , [10] because negative δ 13 C excursions are associated with massive inputs of mantle-derived volcanic CO 2 or the dissolution of methane hydrates, both of which induce global warming. In fact, other OAEs, such as the Toarcian OAE and OAE 1a, were accompanied by prominent negative δ 13 C excursions at their bases [28] , [29] . In case of OAE2, despite evidence of massive volcanic activity and an increase in p CO 2 immediately before OAE2 (refs 5 , 6 , 7 , 8 , 10 ), no prominent negative δ 13 C excursions have been confirmed close to the base of OAE2 at all of the studied sites (except for the Italian section) [10] . Although a negative δ 13 C excursion below the first build-up phase has been reported previously [30] , [31] , the excursion was considered to be a diagenetic signal, or a reflection of local oceanographic episodic events, such as fresh water input. Our results identified a negative δ 13 C wood excursion just below the first build-up phase from two distant sections of the GVS and YG, which is the same excursion reported immediately below the OAE2 horizon in YG sediments in the Kotanbetsu area of northwestern Hokkaido [32] . This evidence suggests the occurrence of a negative shift in the carbon-isotope composition of global atmosphere and/or the change in global terrestrial climate and hydrological cycles immediately before the onset of OAE2. Assuming constant sedimentation rates at these two distant sections, the negative shift began 23–51 ky before the onset of the first build-up phase of OAE2, which is generally consistent with the onset of the volcanic pulse manifested by the negative 187 Os/ 188 Os shift [7] and increased p CO 2 levels [5] . The negative δ 13 C wood excursion in the two Pacific sections may reflect the mass emission of volcanic CO 2 containing isotopically light carbon and/or changes in the terrestrial climate or vegetation that arose because of increased p CO 2 . It has previously been shown that the predominant marine signature around the OAE2 interval in the sections of the Tethys Sea and Atlantic Ocean are the black shales [33] , and that the anoxic environments in these oceans expanded from the photic zone to a depth of more than 3,500 m (refs 3 , 4 ) during OAE2. DOP analysis of the GVS and YG strata revealed several occurrences of very short-term dysoxic conditions (DOP>0.45) in the northeastern and northwestern Pacific ( Fig. 2 ). However, most of the OAE2 intervals of these strata are characterized by low DOP values and the presence of bioturbation and benthic foraminifera throughout the sequences. Even at higher DOP horizons, DOP values are usually <0.75 and bioturbation and benthic foraminifera have a continuous distribution. Therefore, our results indicate that oxic conditions were prevalent at even the upper bathyal depths, which were associated with the development of OMZ [18] in the northeastern and northwestern Pacific Ocean throughout most of the OAE2 interval. Similar studies on shallow water carbonates in the equatorial western Pacific have found no evidence of anoxic conditions during OAE2 (ref. 30 ), which implies that the occurrence of the oceanographic conditions that are conducive to the development of anoxic environments are unlikely to have arisen along the continental margin of Pacific Ocean during OAE2. Sampling procedure The OAE2 interval was studied in the Budden Canyon Formation comprising the GVS that crops out along the North Fork Cottonwood Creek in Shasta County in central California, USA, and the lower part of the Saku Formation of the YG, exposed along the Hakkin River in the Oyubari area of central Hokkaido, Japan. Approximately 130 mudstone samples from the GVS and 250 mudstone and muddy sandstone samples from the YG were collected at 0.3- to 5-m-stratigraphic intervals. Dry sample aliquots of 400 g were disaggregated using sodium tetraphenylborate plus sodium chloride. The disaggregated sediment was washed over a 64-μm sieve and dried at 50 °C. Foraminiferal specimens (all) and wood fragments (more than 100 fragments per sample) were then removed from the processed samples. Nannofossils were viewed using simple smear slide preparations. Carbon isotopes Collected wood fragments, usually more than 100 per sample, were washed in methanol in an ultrasonic bath before immersion in 1 N HCl acid for 24 h. The wood fragments were then dried and crushed to powder and the carbon isotope of the TOC in the acid-treated powdered wood samples was then measured using a mass spectrometer (IsoPrime, GV Instruments) in line with an elemental analyzer (EuroEA3000, EuroVector). Each sample was run in duplicate and carbon-isotopic ratios were expressed in ‰, relative to the Vienna Pee Dee Belemnite standard. The precision of the δ 13 C measurements was ±0.1‰. Definition of the OAE2 interval is based on the 'least conservative estimate of OAE2 (from base of Sciponoceras gracile to Vascoceras birchbyi ammonoid zones)' in ref. 19 . Degree of pyritization Total sulphur content was measured by the dry combustion method using an elemental analyzer (EuroEA3000, EuroVector) at Okayama University. The reactive part of Fe was extracted following method of ref. 34 , by mixing 100 mg of finely ground sample with 5 ml of 1 N HCl for 24 h. Measurements were determined using Inductively Coupled Plasma Atomic Emission Spectrometry (ICPS-8100, Shimadzu) at the Hokkaido Industrial Research Institute. The DOP was calculated using the equation DOP=Fe pyrite /(Fe pyrite +Fe reactive ). Pyrite bound Fe (Fe pyrite ) was approximated by multiplying the S content by 0.871. Sedimentation rate Calculation of mean sedimentation rates of the GVS and YG during OAE2 used two stratigraphic horizons; the base of first build-up and the top of the recovery phases. The thicknesses between these two horizons were divided by the 847–885 ky, which was estimated to be the minimum and maximum duration of δ 13 C excursion during OAE2 at the stratotype section of the base of the Turonian (ref. 19 ). How to cite this article: Takashima R. et al . Prevailing oxic environments in the Pacific Ocean during the mid-Cretaceous Oceanic Anoxic Event 2. Nat. Commun. 2:234 doi: 10.1038/ncomms1233 (2011).